A Ca2+-dependent signalling circuit regulates influenza A virus internalization and infection Various viruses enter host cells via endocytosis, but the molecular mechanisms underlying the specific internalization pathways remain unclear. Here we show that influenza A viruses (IAVs) enter cells via redundant pathways of clathrin-mediated and clathrin-independent endocytosis, with intracellular Ca 2+ having a central role in regulation of both pathways by activating a signalling axis comprising RhoA, Rho-kinase, phosphatidylinositol 4-phosphate 5-kinase (PIP5K) and phospholipase C (PLC). IAV infection induces oscillations in the cytosolic Ca 2+ concentration of host cells, the prevention of which markedly attenuates virus internalization and infection. The small GTPase RhoA is found both to function downstream of the virus-induced Ca 2+ response and itself to induce Ca 2+ oscillations in a manner dependent on Rho-kinase and subsequent PIP5K-PLC signalling. This signalling circuit regulates both clathrin-mediated and clathrin-independent endocytosis during virus infection and seems to constitute a key mechanism for regulation of IAV internalization and infection. Influenza A virus (IAV) is an enveloped virus with a segmented negative-strand RNA genome, which infects a wide variety of birds and mammals. IAV infection is a complex, multistep process. In the initial step (adsorption), the virus attaches to a host cell through binding of its major surface protein, haemagglutinin (HA), to sialylated cell surface proteins. In the second step (internalization or entry), the adhered viral particle enters the cell as a result of invagination of the surface membrane and is delivered from the endocytic vesicle to early endosomes. Finally, in late endosomes, the virus fuses with the endosomal membrane and thereby releases its genome into the cytosol for replication of viral genes and the production of viral components [1] . Clathrin-mediated endocytosis (CME), the most well-characterized endocytic pathway, is the major route of IAV internalization [2] , [3] . Live cell imaging has thus revealed the de novo formation of clathrin-coated pits at the site of virus attachment [4] and, among the adaptor proteins that contribute to CME, Epsin1 has been found to be required for this process [5] . Recent studies have provided evidence for an alternative pathway of IAV internalization, however. Neither pharmacological inhibition of CME, expression of a dominant-negative form of Eps15, knockdown of Epsin1 nor the introduction of monoclonal antibodies to clathrin was found to inhibit IAV infection [3] , [5] , [6] . In addition, viruses have been found to enter cells simultaneously via non-coated pits as well as via clathrin-coated pits [5] . Nevertheless, the mechanism of this alternative means of cell entry exploited by influenza viruses has remained unclear. We recently showed that Ras-phosphoinositide 3-kinase (PI3K) signalling in the host cell regulates IAV internalization [7] . The binding of Ras to PI3K and subsequent PI3K activation in endosomes regulate clathrin-independent endocytosis (CIE) and IAV internalization through this route. We now investigate the mechanism of Ras activation by IAVs and identify Ca 2+ as a mediator of this event. Moreover, we show that Ca 2+ signalling has an indispensable role in IAV infection, not only through the control of CIE via Ras activation but also through that of CME via mobilization of a novel positive feedback circuit consisting of RhoA, Rho-kinase (ROCK), phosphatidylinositol 4-phosphate 5-kinase (PIP5K), phospholipase C (PLC) and Ca 2+ per se . Ras activation by IAVs is mediated by intracellular Ca 2+ To explore the mechanism by which Ras is activated during IAV infection, we first examined whether intracellular Ca 2+ , one of the upstream regulators of Ras [8] , was increased after infection of mouse embryonic fibroblasts (MEFs) with the A/Puerto Rico/8/34 (H1N1; PR8) virus strain. Yellow Cameleon 3.60 (YC3.60), a Ca 2+ sensor based on Förster resonance energy transfer (FRET) from cyan fluorescent protein (CFP) to yellow fluorescent protein [9] , revealed oscillations in the cytosolic Ca 2+ concentration ([Ca 2+ ] i ) associated with virus infection, albeit with substantial variation in the amplitude and frequency of such oscillations among cells ( Fig. 1a–c ; Supplementary Fig. S1a ). Of note, cells expressing the FRET-based biosensors that had been subjected to the analysis were certainly infected with IAV, as revealed by immunofluorescent labelling of the virus nucleoprotein (NP) ( Supplementary Fig. S1b ; see also Supplementary Fig. S6d ). In MDCK cells, PR8, in addition to histamine or fetal bovine serum (FBS; known factors that increase [Ca 2+ ] i , refs 10 , 11 ), also evoked Ca 2+ oscillations, whereas PBS (solvent of the IAV stock solutions) failed to do so ( Supplementary Fig. S1c–f ). Similar Ca 2+ oscillations could be observed in Cos-1 cells ( Supplementary Fig. S1g ), indicating that IAVs have a potential to elevate Ca 2+ in different cell lines. Given that another viral subtype, A/Aichi/2/68 (H3N2), also evoked [Ca 2+ ] i oscillations ( Supplementary Fig. S1h ), this property did not appear to be restricted to a particular viral strain. 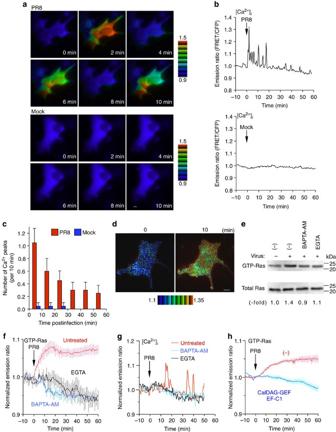Figure 1: Ras activation by IAVs is mediated by intracellular Ca2+. (a–c) MEFs transfected with an expression vector for the FRET-based Ca2+sensor YC3.60 were monitored by dual-emission fluorescence microscopy with exposure to PR8 or mock infection at time 0. FRET/CFP ratio images were generated to represent FRET efficiency, and the upper and lower limits of the ratio range are indicated. Scale bar, 10 μm (a). Representative traces for the FRET/CFP emission ratio (b) and a plot of the number of observed Ca2+peaks versus time averaged for 20 cells (c) are shown. Error bars indicate s.e.m. (d) MEFs expressing Raichu-Ras were monitored by dual-emission fluorescence microscopy with exposure to PR8 at time 0 min. FRET/CFP ratio images at time 0 and 10 min are shown. Scale bar, 10 μm. (e) MEFs were incubated in the absence or presence of 25 μM BAPTA-AM or 1 mM EGTA for 30 min before exposure to PR8 or mock infection. Cell lysates prepared at 0.5 h post-infection (hpi) were subjected to a pull-down assay followed by immunoblot analysis to determine the amount of the active (GTP-bound) form of Ras. An aliquot of cell lysate was also subjected to immunoblot analysis to determine the amounts of total Ras. The intensity of the bands was quantitated by an image analyser, and the fold increase in GTP-bound/total Ras is shown at the bottom. (f,g) MEFs expressing Raichu-Ras (f) or YC3.60 (g) were incubated in the absence or presence of BAPTA-AM or EGTA for 30 min before infection with PR8 at time 0 and were monitored by dual-emission fluorescence microscopy. Normalized emission ratio against time was plotted. Error bars indicate s.e.m. (n=12). (h) Cos-1 cells expressing Raichu-Ras alone or together with the EF-C1 domain of CalDAG-GEFII were infected with PR8 at time 0 and monitored by dual-emission fluorescence microscopy. Normalized emission ratio against time was plotted. Error bars indicate s.e.m. (n=6). Figure 1: Ras activation by IAVs is mediated by intracellular Ca 2+ . ( a – c ) MEFs transfected with an expression vector for the FRET-based Ca 2+ sensor YC3.60 were monitored by dual-emission fluorescence microscopy with exposure to PR8 or mock infection at time 0. FRET/CFP ratio images were generated to represent FRET efficiency, and the upper and lower limits of the ratio range are indicated. Scale bar, 10 μm ( a ). Representative traces for the FRET/CFP emission ratio ( b ) and a plot of the number of observed Ca 2+ peaks versus time averaged for 20 cells ( c ) are shown. Error bars indicate s.e.m. ( d ) MEFs expressing Raichu-Ras were monitored by dual-emission fluorescence microscopy with exposure to PR8 at time 0 min. FRET/CFP ratio images at time 0 and 10 min are shown. Scale bar, 10 μm. ( e ) MEFs were incubated in the absence or presence of 25 μM BAPTA-AM or 1 mM EGTA for 30 min before exposure to PR8 or mock infection. Cell lysates prepared at 0.5 h post-infection (hpi) were subjected to a pull-down assay followed by immunoblot analysis to determine the amount of the active (GTP-bound) form of Ras. An aliquot of cell lysate was also subjected to immunoblot analysis to determine the amounts of total Ras. The intensity of the bands was quantitated by an image analyser, and the fold increase in GTP-bound/total Ras is shown at the bottom. ( f , g ) MEFs expressing Raichu-Ras ( f ) or YC3.60 ( g ) were incubated in the absence or presence of BAPTA-AM or EGTA for 30 min before infection with PR8 at time 0 and were monitored by dual-emission fluorescence microscopy. Normalized emission ratio against time was plotted. Error bars indicate s.e.m. ( n =12). ( h ) Cos-1 cells expressing Raichu-Ras alone or together with the EF-C1 domain of CalDAG-GEFII were infected with PR8 at time 0 and monitored by dual-emission fluorescence microscopy. Normalized emission ratio against time was plotted. Error bars indicate s.e.m. ( n =6). Full size image We further found that Ras activation by IAVs was abolished by chelation of intracellular Ca 2+ with BAPTA-AM, as revealed with both a FRET-based Ras activation sensor [12] and a pull-down assay ( Fig. 1d–g ). In addition, the extracellular Ca 2+ chelator EGTA also inhibited both Ras activation and [Ca 2+ ] i increase by IAVs ( Fig. 1e–g ), demonstrating the requirement for extracellular Ca 2+ in these phenomena. On the other hand, immunoblot analysis with two different antibodies specific for phosphotyrosine (clones 4G10 and PY20) revealed no substantial differences in the tyrosine phosphorylation status of cellular proteins between infected and non-infected cells ( Supplementary Fig. S2a,b ), indicating that IAVs activate Ras via Ca 2+ signalling. Next, to investigate the mechanism(s) through which IAVs induced [Ca 2+ ] i increase and subsequent Ras activation, we prepared virus-like particles (VLPs) from 293T cells transfected with expression vectors for HA, neuraminidase (NA) and matrix protein 1 and 2 (M1 and M2) [13] , [14] . Cell culture media containing VLPs, but not those from mock-transfected 293T cells, induced Ca 2+ oscillations ( Supplementary Fig. S2c ). Sialidase treatment [15] , [16] inhibited Ca 2+ increases by both VLP and PR8 ( Supplementary Fig. S2c,d ), suggesting that attachment of virus particles to sialic acid-containing cell surface molecule(s) has a role in the Ca 2+ elevation. Among Ras activators, a family of Ca 2+ - and diacylglycerol (DAG)-regulated guanine nucleotide exchange factors (CalDAG-GEFs, also known as RasGRPs) [17] , [18] , [19] was a plausible candidate for mediating Ras activation by IAVs, given that this class of GEFs is not only activated by Ca 2+ but also participates in the regulation of Ras in endomembrane compartments including the Golgi apparatus [20] . Expression of the EF-C1 domain of CalDAG-GEFII, which acts in a dominant-negative manner as a result of the absence of the catalytic domain ( Supplementary Fig. S2e ), suppressed virus-induced Ras activation ( Fig. 1h ), but not Ca 2+ oscillations ( Supplementary Fig. S2f ) in Cos-1 cells, implicating CalDAG-GEF as a Ras activator in this pathway. Ca 2+ is a key factor in virus internalization and infection We next evaluated the effect of thapsigargin, an inhibitor of sarcoendoplasmic reticulum Ca 2+ ATPases, on IAV infection. The titre of progeny viruses was markedly increased for MDCK cells treated with thapsigargin at a low dose compared with that for control cells, and dose-dependently reduced at higher doses ( Supplementary Fig. S3a ). Given that thapsigargin raises [Ca 2+ ] i by blocking the sarcoendoplasmic reticulum Ca 2+ ATPases pumps, which thereby causes endoplasmic reticulum stores to become depleted [21] , this result might indicate that intracellular Ca 2+ released from endoplasmic reticulum is crucial for IAV infection and replication. In contrast, BAPTA-AM remarkably reduced the production of progeny viruses ( Fig. 2a ; Supplementary Fig. S3b ). Unexpectedly, given that Ca 2+ was shown to be an upstream regulator of Ras, the inhibitory effect of BAPTA-AM on progeny virus production was much greater than that of the PI3K inhibitor LY294002 ( Fig. 2a ). As LY294002 almost completely inhibited basal and IAV-induced phosphorylation of Akt, the most established downstream molecule of PI3K ( Supplementary Fig. S3c ), it is clear that Ca 2+ also regulates a pathway other than Ras-PI3K signalling. To determine the stage of the virus life cycle at which Ca 2+ signalling is required, we treated cells with BAPTA-AM according to three different regimens: (i) during the early infection stage (from 30 min before infection to 4 h post-infection (hpi)), (ii) during the late stage (from 4 to 24 hpi) and (iii) during both stages. The former two correspond to the periods before and after replication initiation, respectively [7] , [22] ( Supplementary Fig. S3d ). Chelation of Ca 2+ during the early or late stages resulted in a significant reduction in progeny virus production, whereas continuous treatment during both stages inhibited infection to an even greater extent ( Fig. 2b ), suggesting that Ca 2+ functions during both stages. BAPTA-AM treatment during the early stage suppressed infection more efficiently than did LY294002 ( Supplementary Fig. S3e ), again indicative of an effect of Ca 2+ chelation on a viral entry pathway other than Ras-PI3K-dependent CIE. 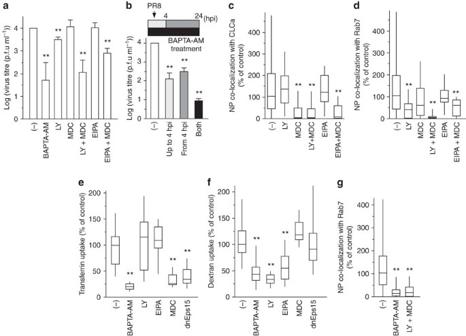Figure 2: Calcium signalling is a key regulator of IAV internalization. (a) MDCK cells were incubated in the absence (−) or presence of 25 μM BAPTA-AM, 50 μM LY294002 (LY), 50 μM MDC or 100 μM EIPA for 30 min before infection with PR8 at a MOI of 1 plaque-forming unit (p.f.u.) per cell for 1 h. The titre of infectious virus particles released into culture supernatants during the continued presence of test agents was determined with an MDCK plaque assay at 48 hpi. Error bars indicate s.d. (n=3). (b) MDCK cells treated with BAPTA-AM according to the indicated regimens and infected with PR8 were evaluated for progeny virus production by the plaque assay at 24 hpi. Error bars indicate s.d. (n=4). (c,d) MDCK cells expressing GFP-tagged clathrin light chain-α (CLCa; c) or GFP-tagged Rab7 (d) were exposed to LY294002, MDC or EIPA for 30 min and infected with PR8 for 1 h. The cells were then fixed, subjected to immunofluorescence staining with antibodies to the virus protein NP and imaged with a confocal microscope. The number of virus particles co-localizing with CLCa- or Rab7-positive vesicles was determined for at least 30 cells in each of three independent experiments and is expressed as a percentage of the corresponding value for control cells in box-and-whisker plots. (e,f) MDCK cells were incubated in the absence or presence of BAPTA-AM, LY, MDC or EIPA for 30 min before exposure to fluorescently labelled transferrin (e) or dextran (f) for 10 min. Cells expressing the dominant-negative form of Eps15 (dnEps15) were also incubated with transferrin or dextran. The uptake of transferrin or dextran was then determined by measurement of fluorescence intensity. Data were obtained for at least 30 cells in each of three independent experiments and are expressed as a percentage of the corresponding value for control cells. (g) Virus internalization for cells treated with BAPTA-AM or with LY294002 and MDC was determined as in d. Data were obtained for at least 30 cells in each of three independent experiments and are expressed as a percentage of the corresponding value for control cells. Inc–g, the highest and lowest boundaries of the box represent the 25th and 75th percentiles, respectively, the whiskers above and below the box designate the 5th and 95th percentiles, respectively, and the line within the box indicates the median value. In all panels, **P<0.01 versus no treatment (−) (Student’st-test). Figure 2: Calcium signalling is a key regulator of IAV internalization. ( a ) MDCK cells were incubated in the absence (−) or presence of 25 μM BAPTA-AM, 50 μM LY294002 (LY), 50 μM MDC or 100 μM EIPA for 30 min before infection with PR8 at a MOI of 1 plaque-forming unit (p.f.u.) per cell for 1 h. The titre of infectious virus particles released into culture supernatants during the continued presence of test agents was determined with an MDCK plaque assay at 48 hpi. Error bars indicate s.d. ( n =3). ( b ) MDCK cells treated with BAPTA-AM according to the indicated regimens and infected with PR8 were evaluated for progeny virus production by the plaque assay at 24 hpi. Error bars indicate s.d. ( n =4). ( c , d ) MDCK cells expressing GFP-tagged clathrin light chain-α (CLCa; c) or GFP-tagged Rab7 ( d ) were exposed to LY294002, MDC or EIPA for 30 min and infected with PR8 for 1 h. The cells were then fixed, subjected to immunofluorescence staining with antibodies to the virus protein NP and imaged with a confocal microscope. The number of virus particles co-localizing with CLCa- or Rab7-positive vesicles was determined for at least 30 cells in each of three independent experiments and is expressed as a percentage of the corresponding value for control cells in box-and-whisker plots. ( e , f ) MDCK cells were incubated in the absence or presence of BAPTA-AM, LY, MDC or EIPA for 30 min before exposure to fluorescently labelled transferrin ( e ) or dextran ( f ) for 10 min. Cells expressing the dominant-negative form of Eps15 (dnEps15) were also incubated with transferrin or dextran. The uptake of transferrin or dextran was then determined by measurement of fluorescence intensity. Data were obtained for at least 30 cells in each of three independent experiments and are expressed as a percentage of the corresponding value for control cells. ( g ) Virus internalization for cells treated with BAPTA-AM or with LY294002 and MDC was determined as in d. Data were obtained for at least 30 cells in each of three independent experiments and are expressed as a percentage of the corresponding value for control cells. In c – g , the highest and lowest boundaries of the box represent the 25th and 75th percentiles, respectively, the whiskers above and below the box designate the 5th and 95th percentiles, respectively, and the line within the box indicates the median value. In all panels, ** P <0.01 versus no treatment (−) (Student’s t -test). Full size image Influenza viruses enter cells via both CME and CIE [5] , [6] , [7] , and recent reports have broadened their entry pathway to macropinocytosis [23] , [24] . To examine the relations among Ca 2+ , endocytosis and virus infection, we established an assay system based on imaging techniques to directly visualize internalized virus particles and evaluate virus internalization at a single-cell level ( Supplementary Fig. S4a,b ). The time course of the number of visualized virus particles and their co-localization with Rab7 (a late endosome marker) was consistent with that obtained by immunoblotting with an anti-M1 antibody ( Supplementary Fig. S3d ) and a previous report [25] . In addition, it could be clarified that virus internalization was dramatically abrogated with the inhibition of endocytosis at 4 °C ( Supplementary Fig. S4c,d ); the established analysis was therefore rational and utilized hereafter. Monodansylcadaverine (MDC), an inhibitor of CME [26] , attenuated virus internalization by the CME pathway ( Fig. 2c ), but it did not affect total virus internalization ( Fig. 2d ) under conditions where CME was dramatically suppressed ( Fig. 2e ). Influenza viruses thus enter host cells via the CIE pathway, including macropinocytosis, even when CME is inhibited, as has been shown previously [5] , [6] , [7] , [27] , [28] . Indeed, MDC had no effect on overall virus infection ( Fig. 2a ; Supplementary Fig. S5a ). A similar inhibitory profile was displayed in cells expressing the dominant-negative mutant of Eps15 (dnEps15, Fig. 2e,f ; Supplementary Fig. S5a,b ), a critical regulator of CME [6] . Suppression of CIE by the PI3K inhibitor LY294002 (ref. 7 ; Fig. 2f ) resulted in only a partial reduction in overall infection ( Fig. 2a ; Supplementary Fig. S5a ). In addition, treatment with the inhibitor of macropinocytosis 5-( N -ethyl- N -isopropyl)-amiloride (EIPA) [29] caused no significant reduction in IAV infection ( Fig. 2a ) under the condition where dextran uptake was suppressed ( Fig. 2f ). Simultaneous inhibition of both CME and CIE (or macropinocytosis), however, resulted in suppression of virus internalization ( Fig. 2d ) and infection ( Fig. 2a ) to an extent greater than that observed with inhibition of either pathway alone. Treatment with BAPTA-AM inhibited both CME and CIE, as evaluated by measurement of the uptake of transferrin ( Fig. 2e ) and dextran ( Fig. 2f ), respectively. Moreover, Ca 2+ chelation inhibited virus internalization ( Fig. 2g ; Supplementary Fig. S5c ) and infection ( Fig. 2a ; Supplementary Fig. S5a ) to an extent similar to that apparent with combined treatment with MDC and LY294002 or MDC and EIPA. Altogether, these results indicate that Ca 2+ signalling is required for both CME- and CIE-mediated virus internalization and that simultaneous inhibition of both these pathways is an effective strategy to block influenza virus infection. Such inhibition can be achieved by combined treatment with MDC and LY294002 (or EIPA) or by treatment with BAPTA-AM alone. Further, this effect of BAPTA-AM was also manifested in both Cos-1 cells and A549 human lung cancer cells ( Supplementary Fig. S5d,e ), indicating that Ca 2+ is generally required for virus internalization in a cell type-independent manner. RhoA and Rac1 activation during IAV infection We next investigated the downstream effectors of Ca 2+ signalling that regulate endocytosis. Given that GTPases of the Rho family are thought to have important roles in vesicular trafficking and to act downstream of Ca 2+ (refs 30 , 31 ), we examined the possible contribution of these proteins to virus internalization. Expression of a dominant-negative mutant (N19) of RhoA resulted in marked inhibition of virus infection and internalization in MDCK cells, whereas that of wild-type RhoA enhanced both infection and internalization ( Fig. 3a,b ; Supplementary Fig. S6a ). Expression of a constitutively active form (V14) of RhoA also inhibited virus infection and internalization, indicating a requirement for the GTP-GDP cycle of RhoA. Whereas RhoA activation by IAVs was not detected with a pull-down assay ( Fig. 3c ; Supplementary Fig. S6b ), it was detected, albeit in a restricted region at the peripheral cell membrane ( Fig. 3d ; Supplementary Fig. S6c ), with the use of a FRET-based RhoA activation sensor [32] . Here it might also be worth mentioning that the FRET-based biosensors utilized in this study did not inhibit IAV infection ( Supplementary Fig. S6d ). 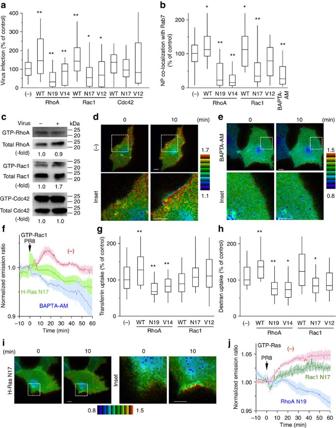Figure 3: Virus internalization is regulated by Rho-family GTPases. (a) MDCK cells were transfected with expression vectors for wild-type (WT) or mutant forms of Rho-family GTPases, or with a control vector (−), incubated with PR8 for 4 h and then fixed and subjected to immunofluorescence with antibodies to NP. Cells expressing the exogenous proteins were identified by expression of ExRed from the bicistronic vectors. Data were obtained for at least 30 cells in each of three independent experiments. *P<0.05, **P<0.01 versus control cells (Student’st-test). (b) MDCK cells expressing GFP-Rab7 and the indicated Rho-family GTPases were infected with PR8 and evaluated for virus internalization. Cells exposed to 25 μM BAPTA-AM for 30 min before PR8 infection were similarly analysed. *P<0.05, **P<0.01 versus control cells (Student’st-test,n=30). (c) Cos-1 cells infected with PR8 for 5 min or subjected to mock infection were lysed and subjected to a pull-down assay. The intensity of the bands was quantitated by an image analyser and the fold increase in GTP-bound/total GTPases is shown at the bottom. (d,e) Cos-1 cells expressing Raichu-RhoA were incubated with BAPTA-AM for 30 min (e) or left untreated (d) before infection with PR8 at time 0 and were subjected to time-lapse microscopy. Scale bars, 10 μm. (f) Cos-1 cells were transfected with an expression vector for Raichu-Rac1 alone or together with a vector for a dominant-negative mutant of Ras (H-Ras N17), incubated with or without BAPTA-AM for 30 min and then infected with PR8 (at time 0). The normalized FRET/CFP emission ratio was plotted. Error bars indicate s.e.m. (g,h) MDCK cells expressing the indicated Rho-family GTPases were subjected to endocytic assays with transferrin (g) or dextran (h) *P<0.05, **P<0.01 versus control cells (Student’st-test,n=30). (i) Cos-1 cells expressing Raichu-RhoA and H-Ras N17 were infected with PR8 at time 0 and subjected to FRET imaging. Scale bar, 10 μm. (j) Cos-1 cells expressing Raichu-Ras alone or together with dominant-negative mutants of RhoA or Rac1 were infected with PR8 at time 0 and subjected to FRET imaging. The normalized FRET/CFP emission ratio was plotted. Error bars indicate s.e.m. Ina,b,gandh, the boundaries of the box, the whiskers above and below the box and the line within the box represent the 25th and 75th percentiles, the 5th and 95th percentiles and the median value, respectively. Figure 3: Virus internalization is regulated by Rho-family GTPases. ( a ) MDCK cells were transfected with expression vectors for wild-type (WT) or mutant forms of Rho-family GTPases, or with a control vector (−), incubated with PR8 for 4 h and then fixed and subjected to immunofluorescence with antibodies to NP. Cells expressing the exogenous proteins were identified by expression of ExRed from the bicistronic vectors. Data were obtained for at least 30 cells in each of three independent experiments. * P <0.05, ** P <0.01 versus control cells (Student’s t -test). ( b ) MDCK cells expressing GFP-Rab7 and the indicated Rho-family GTPases were infected with PR8 and evaluated for virus internalization. Cells exposed to 25 μM BAPTA-AM for 30 min before PR8 infection were similarly analysed. * P <0.05, ** P <0.01 versus control cells (Student’s t -test, n =30). ( c ) Cos-1 cells infected with PR8 for 5 min or subjected to mock infection were lysed and subjected to a pull-down assay. The intensity of the bands was quantitated by an image analyser and the fold increase in GTP-bound/total GTPases is shown at the bottom. ( d , e ) Cos-1 cells expressing Raichu-RhoA were incubated with BAPTA-AM for 30 min ( e ) or left untreated ( d ) before infection with PR8 at time 0 and were subjected to time-lapse microscopy. Scale bars, 10 μm. ( f ) Cos-1 cells were transfected with an expression vector for Raichu-Rac1 alone or together with a vector for a dominant-negative mutant of Ras (H-Ras N17), incubated with or without BAPTA-AM for 30 min and then infected with PR8 (at time 0). The normalized FRET/CFP emission ratio was plotted. Error bars indicate s.e.m. ( g , h ) MDCK cells expressing the indicated Rho-family GTPases were subjected to endocytic assays with transferrin ( g ) or dextran ( h ) * P <0.05, ** P <0.01 versus control cells (Student’s t -test, n =30). ( i ) Cos-1 cells expressing Raichu-RhoA and H-Ras N17 were infected with PR8 at time 0 and subjected to FRET imaging. Scale bar, 10 μm. ( j ) Cos-1 cells expressing Raichu-Ras alone or together with dominant-negative mutants of RhoA or Rac1 were infected with PR8 at time 0 and subjected to FRET imaging. The normalized FRET/CFP emission ratio was plotted. Error bars indicate s.e.m. In a , b , g and h , the boundaries of the box, the whiskers above and below the box and the line within the box represent the 25th and 75th percentiles, the 5th and 95th percentiles and the median value, respectively. Full size image VLPs also activated RhoA at the cell periphery ( Supplementary Fig. S7a ) and both PR8- and VLP-induced RhoA activation was inhibited by BAPTA-AM ( Fig. 3e ; Supplementary Fig. S7a,d ), consistent with the notion that RhoA is activated downstream of Ca 2+ in a spatiotemporally dependent manner. Similarly, expression of dominant-negative (N17) or constitutively active (V12) forms of Rac1 also inhibited virus infection or internalization ( Fig. 3a,b ; Supplementary Fig. S6a ), with IAV-induced activation of Rac1 being detected with both pull-down and FRET-based [33] assays ( Fig. 3c,f ) and being inhibited by BAPTA-AM ( Fig. 3f ; Supplementary Fig. S7b ). In contrast, expression of dominant-negative (N17) or constitutively active (V12) variants of Cdc42 had no significant effect on virus infection ( Fig. 3a ; Supplementary Fig. S6a ), and no marked activation of Cdc42 by IAVs was observed with pull-down ( Fig. 3c ) or FRET ( Supplementary Fig. S7c ) assays. These results thus indicate that Cdc42 is dispensable for influenza virus infection. We also examined the effects of exogenous RhoA or Rac1 expression on endocytosis in MDCK cells. The uptake of both transferrin and dextran was enhanced by wild-type RhoA and inhibited by its dominant-negative mutant ( Fig. 3g,h ), indicating that RhoA promotes both CME and CIE. On the other hand, Rac1 expression affected only the uptake of dextran ( Fig. 3g,h ), suggesting that Rac1 regulates CIE but not CME, consistent with previous observations [34] , [35] . We examined the molecular hierarchy among RhoA, Rac1 and Ras. Activation of Rac1, but not that of RhoA, was inhibited by expression of a dominant-negative form (N17) of H-Ras ( Fig. 3f,i ; Supplementary Fig. S7d ). Further, expression of the dominant-negative form of RhoA suppressed IAV-dependent Ras activation, whereas that of the dominant-negative form of Rac1 did not ( Fig. 3j ). These results thus indicate that RhoA acts upstream of Ras and Rac1, and that Rac1 functions downstream of Ras. RhoA promotes Ca 2+ oscillations Unexpectedly, we noticed that RhoA also acts as an upstream regulator of Ca 2+ . Expression of the dominant-negative variant of RhoA in Cos-1 and MDCK cells prevented the infection-evoked [Ca 2+ ] i oscillations observed in control cells, whereas the expression of wild-type RhoA increased the frequency of such oscillations ( Fig. 4a ; Supplementary Fig. S8a ). Expression of Rac1 did not affect virus-induced Ca 2+ oscillation ( Fig. 4a ), indicating that the reciprocal regulatory relation between RhoA and Ca 2+ is specific. Substantial Ca 2+ oscillations were also apparent in cells expressing wild-type RhoA before virus infection ( Fig. 4a ). Indeed, both wild-type and constitutively active forms of RhoA, but not Rac1 or Cdc42, induced Ca 2+ oscillation in the absence of extracellular stimuli, the amplitudes and frequencies of which differed among cell lines ( Fig. 4b ; Supplementary Fig. S8b ). These observations therefore suggested that GTP-RhoA and Ca 2+ constitute a positive feedback loop, with RhoA not only being activated by Ca 2+ but also inducing subsequent [Ca 2+ ] i elevation during virus infection. 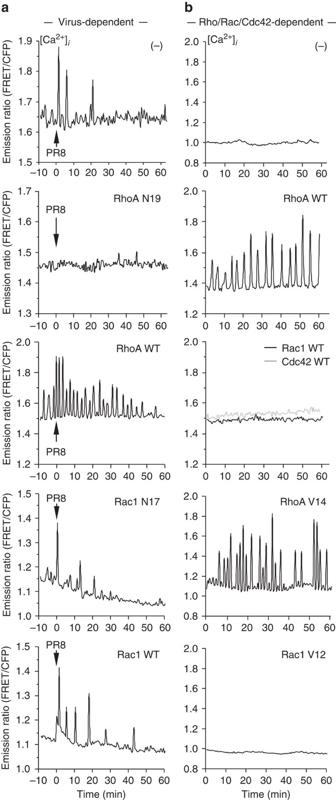Figure 4: RhoA enhances virus-induced Ca2+oscillations. (a) Cos-1 cells were transfected for 24 h with expression vectors for YC3.60 and either wild-type (WT) or dominant-negative forms of RhoA or Rac1, as indicated, infected with PR8 (at time 0) and subjected to time-lapse fluorescence microscopy. IAV-induced oscillations in cells expressing YC3.60 alone is shown as a control. (b) Cos-1 cells expressing YC3.60 and either WT or constitutively active forms of RhoA, Rac1 or Cdc42 were observed by fluorescence microscopy to monitor [Ca2+]i. The transition of [Ca2+]iof cells expressing YC3.60 alone is shown as a control. Figure 4: RhoA enhances virus-induced Ca 2+ oscillations. ( a ) Cos-1 cells were transfected for 24 h with expression vectors for YC3.60 and either wild-type (WT) or dominant-negative forms of RhoA or Rac1, as indicated, infected with PR8 (at time 0) and subjected to time-lapse fluorescence microscopy. IAV-induced oscillations in cells expressing YC3.60 alone is shown as a control. ( b ) Cos-1 cells expressing YC3.60 and either WT or constitutively active forms of RhoA, Rac1 or Cdc42 were observed by fluorescence microscopy to monitor [Ca 2+ ] i . The transition of [Ca 2+ ] i of cells expressing YC3.60 alone is shown as a control. Full size image Requirement for PIP5K in virus internalization and infection PIP5K has been shown to regulate endocytosis [36] , [37] downstream of Rho-family GTPases [38] . We examined the role of PIP5K in the regulation of CME and CIE with the use of MEFs isolated from wild-type and PIP5Kα-deficient (PIP5K −/− ) mice [39] . The uptake of both transferrin and dextran was reduced in PIP5K −/− MEFs compared with that in wild-type cells ( Fig. 5a,b ), as were the internalization ( Fig. 5c ) and progeny production of IAVs ( Fig. 5d ). Further, virus-dependent [Ca 2+ ] i oscillations were reduced in frequency and delayed in PIP5K-deficient cells compared with those in wild-type cells ( Fig. 5e–h ). 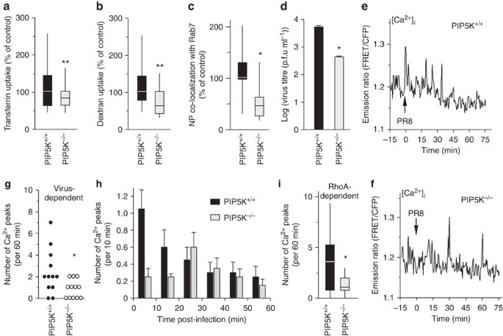Figure 5: Role of PIP5K in virus internalization. (a,b) Wild-type or PIP5K-deficient MEFs were assayed for the uptake of transferrin (a) or dextran (b). **P<0.01 versus wild-type (control) cells. (Student’st-test,n=20). (c) MEFs expressing GFP-Rab7 were infected with PR8 and evaluated for virus internalization. *P<0.05 versus wild-type cells (Student’st-test,n=30). (d) MEFs were infected with PR8 at an MOI of 1 p.f.u. per cell for 1 h, and the titre of infectious virus particles released into culture supernatants during the subsequent 2 days was determined with an MDCK plaque assay. Data are means±s.d. from three independent experiments. *P<0.05 versus wild-type cells (Student’st-test,n=3). (e–h) Wild-type (e) and PIP5K−/−(f) MEFs expressing YC3.60 were infected with PR8 at time 0 and were observed by fluorescence microscopy to monitor [Ca2+]i. The number of Ca2+peaks observed between time 0 and 60 min in individual cells was determined (g). The observation period was also divided into six 10-min intervals, and the number of observed Ca2+peaks in each interval was counted and averaged for 20 cells (h). Error bars indicate s.e.m. (i) Wild-type and PIP5K-deficient MEFs expressing YC3.60 and wild-type RhoA were processed as in g. *P<0.05 versus wild-type cells (Student’st-test,n=45). Ina–candi, the boundaries of the box, the whiskers above and below the box and the line within the box represent the 25th and 75th percentiles, the 5th and 95th percentiles and the median value, respectively. Figure 5: Role of PIP5K in virus internalization. ( a , b ) Wild-type or PIP5K-deficient MEFs were assayed for the uptake of transferrin ( a ) or dextran ( b ). ** P <0.01 versus wild-type (control) cells. (Student’s t -test, n =20). ( c ) MEFs expressing GFP-Rab7 were infected with PR8 and evaluated for virus internalization. * P <0.05 versus wild-type cells (Student’s t -test, n =30). ( d ) MEFs were infected with PR8 at an MOI of 1 p.f.u. per cell for 1 h, and the titre of infectious virus particles released into culture supernatants during the subsequent 2 days was determined with an MDCK plaque assay. Data are means±s.d. from three independent experiments. * P <0.05 versus wild-type cells (Student’s t -test, n =3). ( e – h ) Wild-type ( e ) and PIP5K −/− ( f ) MEFs expressing YC3.60 were infected with PR8 at time 0 and were observed by fluorescence microscopy to monitor [Ca 2+ ] i . The number of Ca 2+ peaks observed between time 0 and 60 min in individual cells was determined ( g ). The observation period was also divided into six 10-min intervals, and the number of observed Ca 2+ peaks in each interval was counted and averaged for 20 cells ( h ). Error bars indicate s.e.m. ( i ) Wild-type and PIP5K-deficient MEFs expressing YC3.60 and wild-type RhoA were processed as in g. * P <0.05 versus wild-type cells (Student’s t -test, n =45). In a – c and i , the boundaries of the box, the whiskers above and below the box and the line within the box represent the 25th and 75th percentiles, the 5th and 95th percentiles and the median value, respectively. Full size image Next, we examined whether IAVs and RhoA indeed activated PIP5K. PIP5K is reported to be tyrosine-phosphorylated and unphosphorylated in its inactive and active forms, respectively, the difference between which can be distinguished by the electrophoretic mobility shift [40] . The slower migrating fractions of PIP5K were decreased on PR8 infection in a time-dependent manner ( Supplementary Fig. S9a ), and by expression of wild type and the activated mutant of RhoA, whereas its dominant-negative mutant failed to do so ( Supplementary Fig. S9b ). In addition, both PR8 and wild-type RhoA promoted the translocation of PIP5K from the cytoplasm to the plasma membrane and the Golgi ( Supplementary Fig. S9c ), where PIP5K is known to be activated [41] , whereas expression of dominant-negative form of RhoA suppressed PR8-induced PIP5K translocation. Further, RhoA-dependent Ca 2+ oscillations were substantially suppressed in PIP5K −/− cells ( Fig. 5i ), indicating that RhoA-dependent PIP5K activation modulates IAV-induced Ca 2+ signalling. ROCK as an adaptor bridging RhoA and PIP5K Given that ROCK has an important role in RhoA-PIP5K signalling [38] , [42] , we investigated whether ROCK participates in the regulation of IAV-induced Ca 2+ signalling. The ROCK inhibitor Y-27632 (ref. 43 ) did not affect CME or CIE in MDCK cells ( Supplementary Fig. S10a,b ). Moreover, whereas BAPTA-AM suppressed RhoA-induced Ca 2+ oscillations, Y-27632 failed to do so ( Fig. 6a,b ), although it disrupted the organization of actin stress fibres ( Supplementary Fig. S10c ). These results thus suggested that the kinase activity of ROCK is dispensable for endocytosis and RhoA-induced Ca 2+ signalling. Instead, CIE seemed to be inhibited by excess activation of ROCK, given that Y-27632 reversed the inhibitory effect of the constitutively active mutant of RhoA on dextran uptake ( Supplementary Fig. S10d ). RhoA has been shown to interact directly with PIP5K irrespective of the bound nucleotide [41] , [44] . To further confirm the requirement for activated RhoA in an IAV-dependent Ca 2+ signalling, we made use of the Rho-binding domain (RBD) of ROCK1, which, through the trapping of GTP-RhoA, exerts a dominant-negative effect on its downstream effectors including ROCK [45] . Expression of the RBD suppressed virus-dependent and RhoA-dependent Ca 2+ oscillations ( Fig. 6c,d ), endocytic activity ( Supplementary Fig. S10e,f ) as well as virus infection and internalization ( Fig. 6e,f ; Supplementary Fig. S10g ). These results indicated that RhoA mediates virus-evoked signalling in a manner dependent on its binding of GTP. 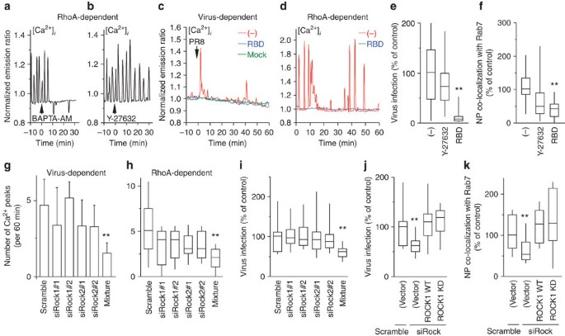Figure 6: ROCK mediates RhoA signalling during IAV infection in a manner independent of its kinase activity. (a,b) Cos-1 cells expressing YC3.60 and wild-type RhoA were exposed to BAPTA-AM (a) or Y-27632 (b) at time 0 and observed by fluorescence microscopy. (c,d) Cos-1 cells expressing YC3.60 alone or together with the RBD of ROCK1 were either infected with PR8 at time 0 (c) or transfected with a vector for wild-type RhoA (d), and were monitored for [Ca2+]i. (e,f) Cos-1 cells were transfected for 24 h with an expression vector for the RBD of ROCK1 or a control vector, and were then incubated in the absence or presence of Y-27632 for 30 min. Virus infection (e) and internalization (f) were then evaluated. **P<0.01 versus control cells (Student’st-test,n=20). (g,h) MEFs were transfected with siRNAs (#1 or #2) specific for ROCK1 or ROCK2 messenger RNAs or with a scrambled siRNA for 48 h, and were then further transfected for 24 h with an expression vector encoding YC3.60 (g) or with vectors for YC3.60 and wild-type RhoA (h). Ing, the cells were infected with PR8 at time 0. The numbers of Ca2+peaks observed in individual cells over 60 min were counted. Error bars indicate s.d. ‘Mixture’ indicates that cells were transfected with all four ROCK siRNAs. **P<0.01 versus control cells (Student’st-test,n=10). (i) Cells transfected with ROCK siRNAs as ingwere subjected to a virus infection assay. **P<0.01 versus control cells (Student’st-test, n=20). (j,k) MEFs were transfected with all four ROCK siRNAs (siRock) or a scrambled siRNA for 48 h and were then further transfected for 24 h with an expression vector for wild-type (WT) or kinase-dead (KD) forms of human ROCK1, or an empty vector (control). Ink, an expression vector for GFP-Rab7 was also introduced during a second transfection step. Virus infection (j) and internalization (k) were then evaluated. **P<0.01 versus control cells (Student’st-test,n=20). Ine,fandh–k, the boundaries of the box, the whiskers above and below the box and the line within the box represent the 25th and 75th percentiles, the 5th and 95th percentiles and the median value, respectively. Figure 6: ROCK mediates RhoA signalling during IAV infection in a manner independent of its kinase activity. ( a , b ) Cos-1 cells expressing YC3.60 and wild-type RhoA were exposed to BAPTA-AM ( a ) or Y-27632 ( b ) at time 0 and observed by fluorescence microscopy. ( c , d ) Cos-1 cells expressing YC3.60 alone or together with the RBD of ROCK1 were either infected with PR8 at time 0 ( c ) or transfected with a vector for wild-type RhoA ( d ), and were monitored for [Ca 2+ ] i . ( e , f ) Cos-1 cells were transfected for 24 h with an expression vector for the RBD of ROCK1 or a control vector, and were then incubated in the absence or presence of Y-27632 for 30 min. Virus infection ( e ) and internalization ( f ) were then evaluated. ** P <0.01 versus control cells (Student’s t -test, n =20). ( g , h ) MEFs were transfected with siRNAs (#1 or #2) specific for ROCK1 or ROCK2 messenger RNAs or with a scrambled siRNA for 48 h, and were then further transfected for 24 h with an expression vector encoding YC3.60 ( g ) or with vectors for YC3.60 and wild-type RhoA ( h ). In g , the cells were infected with PR8 at time 0. The numbers of Ca 2+ peaks observed in individual cells over 60 min were counted. Error bars indicate s.d. ‘Mixture’ indicates that cells were transfected with all four ROCK siRNAs. ** P <0.01 versus control cells (Student’s t -test, n =10). ( i ) Cells transfected with ROCK siRNAs as in g were subjected to a virus infection assay. ** P <0.01 versus control cells (Student’s t -test, n=20). ( j , k ) MEFs were transfected with all four ROCK siRNAs (siRock) or a scrambled siRNA for 48 h and were then further transfected for 24 h with an expression vector for wild-type (WT) or kinase-dead (KD) forms of human ROCK1, or an empty vector (control). In k , an expression vector for GFP-Rab7 was also introduced during a second transfection step. Virus infection ( j ) and internalization ( k ) were then evaluated. ** P <0.01 versus control cells (Student’s t -test, n =20). In e , f and h – k , the boundaries of the box, the whiskers above and below the box and the line within the box represent the 25th and 75th percentiles, the 5th and 95th percentiles and the median value, respectively. Full size image We then revisited the relevance of ROCK to GTP-RhoA-mediated PIP5K activation by depleting MEFs of endogenous ROCK through transfection with specific short interfering RNAs (siRNAs). The knockdown efficiencies for ROCK1 and ROCK2 with corresponding siRNAs were ~70% and ~30%, respectively ( Supplementary Fig. S11a,b ). Knockdown of ROCK1 or ROCK2 alone resulted in partial inhibition of both IAV- and RhoA-dependent Ca 2+ oscillations, whereas the simultaneous knockdown of both proteins resulted in almost complete inhibition ( Fig. 6g,h ; Supplementary Fig. S11c ). Consistent with these results, knockdown of ROCK1 or ROCK2 alone had a minimal effect on IAV infection, whereas simultaneous depletion of both ROCK isoforms effectively reduced infection ( Fig. 6i ). ROCK1 and ROCK2 thus participate in RhoA-mediated PIP5K activation and IAV infection in a manner independent of their kinase activity. This conclusion was further confirmed by the observation that expression of wild-type human ROCK1 or a kinase-defective mutant thereof restored IAV infection and internalization in MEFs depleted of endogenous ROCK1 and ROCK2 ( Fig. 6j,k ). Altogether, our results indicate that RhoA-bound ROCK, but not the kinase activity of ROCK, is essential for RhoA-dependent Ca 2+ signalling and IAV infection. PLC is required for RhoA-dependent Ca 2+ oscillations Finally, we attempted to identify the mechanism by which Ca 2+ signalling is regulated by PIP5K. Given the established role of PLC in the conversion of phosphatidylinositol 4,5-bisphosphate to inositol 1,4,5-trisphosphate (IP3) and DAG, we examined the effect of the PLC inhibitor U73122 (ref. 46 ) on IAV-induced Ca 2+ oscillations. Exposure of Cos-1 cells to U73122 prevented the increase in [Ca 2+ ] i triggered by infection with PR8 ( Fig. 7a ) as well as the spontaneous Ca 2+ oscillations apparent in cells overexpressing wild-type RhoA ( Fig. 7b ). Further, U73122 prevented IAV internalization ( Fig. 7c ), and similar inhibitory profiles could be observed when another PLC inhibitor edelfosine [46] , [47] was utilized ( Supplementary Fig. S12a,b ). In addition, these reagents dramatically inhibited peripheral RhoA activation by PR8 ( Fig. 7d ; Supplementary Fig. S12c compared with Fig. 3d and Supplementary Fig. S6c ). Altogether, our results thus suggest that the positive feedback loop between Ca 2+ and RhoA, which is mediated by ROCK, PIP5K and PLC, governs both CME and CIE, with the latter being regulated by the CalDAG-GEF-Ras-PI3K-Rac1 pathway ( Fig. 8 ). This signalling network provides an acceptor system of host cells for IAV internalization through which IAVs, indeed, activate both CME and CIE to produce a favourable circumstance for their entry ( Supplementary Fig. S13a,b ). 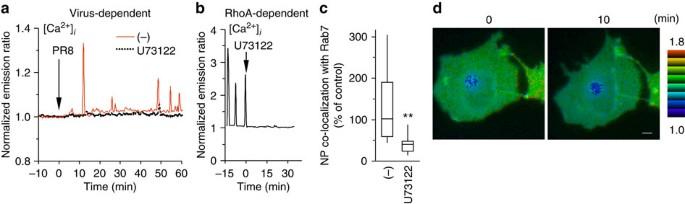Figure 7: PLC participates in the induction of Ca2+oscillations by RhoA. (a) Cos-1 cells expressing YC3.60 were incubated in the absence or presence of 5 μM U73122 for 30 min before infection with PR8 at time 0. The cells were monitored for Ca2+transitions. (b) Cos-1 cells expressing YC3.60 and wild-type RhoA were subjected to Ca2+imaging, with the addition of U73122 at time 0. (c) Cos-1 cells expressing GFP-Rab7 were incubated in the absence or presence of 5 μM U73122 for 30 min and were then infected with PR8 for 1 h. Virus internalization was evaluated. **P<0.01 versus control cells (Student’st-test,n=30) The boundaries of the box, the whiskers above and below the box and the line within the box represent the 25th and 75th percentiles, the 5th and 95th percentiles and the median value, respectively. (d) Cos-1 cells expressing Raichu-RhoA were incubated with U73122 for 30 min before infection with PR8 at time 0. The cells were subjected to time-lapse microscopy to visualize RhoA activation. Scale bar, 10 μm. Figure 7: PLC participates in the induction of Ca 2+ oscillations by RhoA. ( a ) Cos-1 cells expressing YC3.60 were incubated in the absence or presence of 5 μM U73122 for 30 min before infection with PR8 at time 0. The cells were monitored for Ca 2+ transitions. ( b ) Cos-1 cells expressing YC3.60 and wild-type RhoA were subjected to Ca 2+ imaging, with the addition of U73122 at time 0. ( c ) Cos-1 cells expressing GFP-Rab7 were incubated in the absence or presence of 5 μM U73122 for 30 min and were then infected with PR8 for 1 h. Virus internalization was evaluated. ** P <0.01 versus control cells (Student’s t -test, n =30) The boundaries of the box, the whiskers above and below the box and the line within the box represent the 25th and 75th percentiles, the 5th and 95th percentiles and the median value, respectively. ( d ) Cos-1 cells expressing Raichu-RhoA were incubated with U73122 for 30 min before infection with PR8 at time 0. The cells were subjected to time-lapse microscopy to visualize RhoA activation. Scale bar, 10 μm. 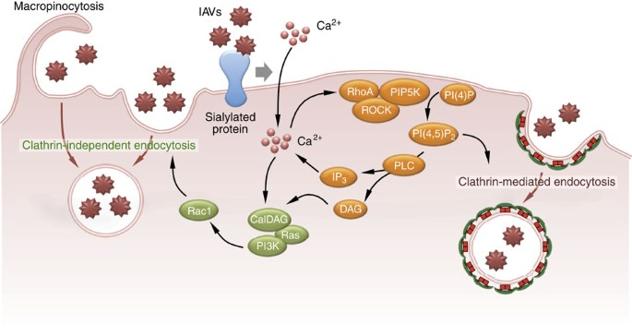Figure 8 Model for the intracellular signalling circuit that underlies the regulation of IAV internalization via CME and CIE. Full size image Figure 8 Model for the intracellular signalling circuit that underlies the regulation of IAV internalization via CME and CIE. Full size image We have shown here that an increase in [Ca 2+ ] i is required for IAV infection and internalization via CIE and CME, and that RhoA, in cooperation with ROCK, PIP5K and PLC, regulates this Ca 2+ signalling and is itself regulated by Ca 2+ . We and others have previously shown that PI3K is required for CIE and influenza virus infection [7] , [22] , and Epsin1 has been found to be required for virus internalization via CME [5] . However, the molecular mechanisms by which influenza viruses exploit CIE and CME for their efficient internalization by host cells have remained unclear. We now unveil the host cell machinery, consisting of Ca 2+ -RhoA-ROCK-PIP5K-PLC and CalDAG-GEFs-Ras-PI3K-Rac1, that contributes this phenomenon ( Fig. 8 ). Intracellular Ca 2+ has previously been implicated in IAV infection [48] , [49] , with Ca 2+ having been thought to have a role in the late stage of infection. For instance, Ca 2+ acting through calmodulin is required for the transcription and replication of IAV genes [48] , [49] , with inhibition of such Ca 2+ action being expected to attenuate viral messenger RNA replication in the nucleus. Consistent with this notion, we found that BAPTA-AM treatment during the late stage of IAV infection inhibited the generation of progeny viruses, albeit less efficiently than that during the early stage. However, we have also unveiled a hitherto unknown function of Ca 2+ in IAV internalization through the regulation of CME and CIE. Indeed, Ca 2+ oscillations were observed immediately after exposure of cells to the virus. Although the precise mechanism by which IAVs induce [Ca 2+ ] i elevation remains obscure, the elimination of Ca 2+ signalling by BAPTA-AM resulted in almost complete inhibition of virus internalization. In addition to this central role of Ca 2+ in IAV infection, Ca 2+ is also implicated in apoptosis of cells infected by a highly pathogenic H5N1 virus [50] , suggesting that the development of agents that target Ca 2+ signalling might provide a new approach to the prevention and treatment of infection with a variety of influenza subtypes. The [Ca 2+ ] i is maintained at a low level under basal conditions, with increases triggering a variety of cellular responses including gene expression and the release of humoral factors [51] , [52] . In most instances, increases in [Ca 2+ ] i occur in the form of oscillations, which are maintained by a sustained increase in IP3 levels [53] . The RhoA-ROCK-PIP5K-PLC pathway identified in the present study probably contributes to the maintenance of IP3 levels and subsequent Ca 2+ oscillations during influenza virus infection. Such Ca 2+ oscillations in turn activate RhoA; through this positive feedback loop, RhoA, in cooperation of Ca 2+ , has indispensable roles for IAV internalization. With progression of internalization and infection, the input signal from the cell surface to any component molecule (possibly an initial Ca 2+ increase via sialylated proteins) becomes attenuated, leading to the consequent decay of the entire signalling circuit in a time-dependent manner, as recorded by time-lapse microscopy. Although growing evidence implicates Ca 2+ in RhoA signalling [54] , [55] , [56] , little has been reported about the factor articulating these two molecules. The activity of small GTPases is regulated by the balance between the activities of GEFs and GTPase-activating proteins. A myriad of the regulators have been identified over the last decades and the largest family of RhoGEFs comprises the Dbl-family RhoGEFs with 70 human members [57] . Coupled with the redundancy in substrate recognition across the GEF family [58] , the diversity and complexity of GTPase regulation may have prevented us from narrowing down the focus to definitive candidates. In fact, as far as we are aware, PDZ-RhoGEF (ARHGEF11) is only a RhoA-specific GEF that links Ca 2+ signalling to RhoA [56] . However, it unlikely contributes to RhoA activation during IAV infection, given that the protein tyrosine kinase Pyk2, a key factor for PDZ-RhoGEF activation by Ca 2+ signalling downstream of G-protein-coupled receptor, has not previously been implicated in influenza virus infection. Further studies, including a search for relevant GTPase-activating proteins, are therefore required to clarify the molecular linkage between Ca 2+ and RhoA, the mechanism for spatiotemporally specific regulation of RhoA and their contribution to subsequent virus infection. The pathway of virus entry into cells, including that of IAVs, is one of the most studied aspects of the viral life cycle [4] , [59] , [60] . Although considerable effort has been devoted to identifying molecules involved in these pathways, simple inhibition of CME or CIE has yielded only partial effects on infection [2] , [3] , [4] , [5] , [7] , [23] , [28] (see also Fig. 2a,d ) or displayed cell-type-specific inhibition [61] . Similarly, the contribution of GTPases, namely Rac1, to the regulation of entry pathways could be varied across cell types or virus strains [23] , [24] . In addition, in the presence of serum, IAVs exploit macropinocytosis, a class of CIE, as a primary entry route ( Supplementary Fig. S5f,g ) [23] . Hence, the bias between CME and CIE exists in a cell context- and condition-dependent manner and, on inhibition of one of these redundant pathways, IAVs tend to switch to the other pathway to achieve internalization. We have now shown that simultaneous inhibition of both CME and CIE (including macropinocytosis) resulted in suppression of IAV infection effectively, suggesting that CME and CIE are the predominant entry pathways for IAVs. Given that the signalling circuit identified in the present study operates at a branch point of CME and CIE, our results may provide a basis for the development of improved strategies for treatment or prevention of IAV infection. Plasmids Expression vectors for GFP-Rab7, GFP-CLCa, GFP-dnEps15 and the FRET-based biosensor YC3.60 (ref. 9 ) were kindly provided by T. Tsuboi (University of Tokyo, Japan), Y. Kawaoka (University of Wisconsin, Madison, USA), A. Dautry-Varsat (the Pasteur Institute, France) and A. Miyawaki (Riken, Wako, Japan), respectively. The complementary DNA for mouse CalDAG-GEFII, expression vectors for wild-type and mutant human GTPases and those for FRET-based GTPase biosensors (Raichu-Ras (146X), Raichu-RhoA (1293X), Raichu-Rac1 (1026X) and Raichu-Cdc42 (1069X)) [12] , [26] , [32] , [33] were kindly provided by M. Matsuda (Kyoto University, Japan). pCAGGS-HA, pCAGGS-NA, pCAGGS-M1 and pCAGGS-M2, vectors for generation of VLPs, were obtained from Y. Kawaoka. Expression plasmids for human ROCK1 or its kinase-dead (KD) mutant and that for GFP-PIP5K, pCAGGS-myc-ROCK1 and pCAGGS-myc-ROCK1-KD were described previously [43] , [62] . The coding sequences for the EF-C1 domain of mouse CalDAG-GEFII and the RBD of human ROCK1 were amplified by PCR, followed by subcloning into the Xho I and Not I sites of the pCAGGS-Flag-IRES-ExRed vector [63] . The vectors for GTPases, the EF-C1 domain of CalDAG-GEFII and the RBD of ROCK1 were bicistronic to allow monitoring of expression on the basis of the fluorescence of the encoded ExRed. Cells and transfection MEFs deficient in PIP5K (PIP5Kα encoded by PIPKIα gene) were prepared from 12.5 days post-coitum mouse embryos as described previously [39] . Briefly, embryos were collected, the brain and internal organs were removed and the carcasses were minced and incubated with trypsin for 30–45 min at 37 °C. DMEM supplemented with 10% FBS was added to the cell suspension and the cells were further disaggregated. Homogeneous cell suspensions were added to 90-mm dishes containing 10 ml of media. MEFs, Cos-1 (JCRB9082), HEK293T (CRL-11268) and A549 (CCL-185) cells were maintained under a humidified atmosphere of 5% CO2 at 37 °C in DMEM supplemented with 10% FBS, whereas MDCK cells (CCL-34) were maintained in MEM medium (Sigma) with 10% FBS. Expression vectors were introduced into MEFs by nucleofection with the use of an Amaxa (Cologne, Germany) instrument (solution V, program T-20). The FuGene HD reagent (Roche) was used for transfection into other cell types. In principle, MEFs and Cos-1 cells were utilized in knockout/knockdown and overexpression experiments, respectively, whereas MDCK cells were used for assessment of endocytosis/virus internalization. A549 was employed as a model for airway epithelial cells. Reagents and antibodies Hoechst 33342, AlexaFluor488- or AlexaFluor546-labelled dextran (10 kDa), AlexaFluor546-labelled transferrin, AlexaFluor 594-conjugated phalloidin and AlexaFluor488-, AlexaFluor594- or AlexaFluor647-conjugated antibodies to mouse immunoglobulin were obtained from Invitrogen (Carlsbad, CA). Platelet-derived growth factor (50 ng ml −1 ), histamine (100 μM) and phorbol 12-myristate 13-acetate (100 nM) were obtained from PeproTech (Rocky Hill, NJ), Nacalai Tesque (Kyoto, Japan) and Sigma (St Louis, MO), respectively. LY294002 (used at 50 μM), Y-27632 (10 μM) and U73122 (5 μM) were obtained from Calbiochem (San Diego, CA), and MDC (50 μM), acetoxymethyl ester of 1,2-bis(2-aminophenoxy)ethane- N , N , N′ , N′ -tetra acetic acid (BAPTA-AM, 25 μM), EIPA (100 μM), sialidase from Vibrio cholerae (5mU ml −1 ) and thapsigargin were from Sigma. Of note, some of the above reagents were employed at a concentration at which ~95% inhibitory effect could be obtained, according to the previous reports (LY294002, 50 μM (ref. 64 ); EIPA, 100 μM (ref. 65 )) or results of our preliminary experiments (MDC, 50 μM; BAPTA-AM, 25 μM; Supplementary Fig. S14 ). Antibodies to Ras (Ab-3) were obtained from Oncogene (Cambridge, MA), those to RhoA (26C4) and β-actin (I-19) were from Santa Cruz Biotechnology (Santa Cruz, CA), those to Cdc42 (#05-542) were from Millipore (Billerica, MA), those to Rac1 (clone 10) were from BD Bioscience (San Diego, CA), those to phospho-Akt (S473), Akt, ROCK1 (C8F7) and ROCK2 were from Cell Signaling (Danvers, MA) and those to IAV M1 (GA2B) were from Abcam (Cambridge, MA). The 4G10 and PY20 antibodies to phosphotyrosine were obtained from Millipore and BD Bioscience, respectively. Antibodies to NP and GFP were kindly provided by A. Takada (Hokkaido University) and M. Matsuda, respectively. Viruses IAV strains PR8 and A/Aichi/2/68 (H3N2) were propagated in the chorioallantoic cavity of 10-day-old embryonated chicken eggs for 48 h at 37 °C. After high-speed centrifugation, the purified viruses were resuspended in PBS buffer and stored at −80 °C until use. Cells were infected with PR8 at a multiplicity of infection (MOI) of 1 p.f.u. per cell at 37 °C. The amount of infectious virus in culture supernatants was determined with a plaque assay as described previously [66] , [67] . Briefly, confluent monolayers of MDCK cells in 12-well plates were inoculated with the supernatants. After 1 h of adsorption, the cell supernatants were removed, and the cells were overlaid with MEM containing 1% Bact-agar and trypsin (5 mg ml −1 ). Plaques were enumerated after incubation at 35 °C and 5% CO2 for 2 days. Generation of VLPs Generation of VLPs was conducted according to the previous report [13] , [14] . Briefly, 293T cells (1 × 10 6 cells) in a 6-cm-diameter dish were transfected with expression vectors for PR8 HA, NA, M1 and M2 and at 6 hpi, the medium was replaced with OPTIMEM (Invitrogen). After 48 h, the culture medium was collected, subjected to centrifugation at 2,000 g for 10 min to remove cell debris and then used for analysis. Culture media obtained from cells transfected with empty vectors were used as a negative control. Immunoblot analysis and pull-down assay for small GTPases Unless otherwise specified, cells were lysed in RIPA buffer (50 mM Tris–HCl (pH 7.4), 150 mM NaCl, 1 mM EDTA, 1% Nonidet P-40, 0.1% SDS, 0.5% sodium deoxycholate, 1 mM Na 3 VO 4 ) for 20 min on ice. For detection of phosphorylated and unphosphorylated PIP5K, Cos-1 cells expressing GFP-PIP5K were infected with PR8 at an MOI of 10 for 0, 30 and 60 min or stimulated with phorbol 12-myristate 13-acetate for 30 min. Cells were lysed in a solution containing 10 mM Tris–HCl, pH 7.4, 150 mM NaCl, 30 mM sodium pyrophosphate, 0.5% Nonidet P-40, 5 mM EDTA, 10% glycerol, 50 mM NaF, 1 mM Na 3 VO 4 , 1 mM phenylmethylsulfonyl fluoride, 10 μg ml −1 aprotinin and 10 μg ml −1 leupeptin for 30 min on ice. The lysates were centrifuged at 20,000 g for 10 min at 4 °C, and the resulting supernatants were subjected to SDS–polyacrylamide gel electrophoresis. The separated proteins were transferred to a polyvinylidene difluoride membrane (Bio-Rad, Hercules, CA) and subjected to immunoblot analysis. Immune complexes were detected with the use of ECL Western Blotting Detection Reagent (GE Healthcare, Little Chalfont, UK) and an LAS-1000UVmini image analyser. Detection of GTP-bound Ras- and Rho-family GTPases was performed essentially as described previously [68] , [69] , with slight modifications [63] , [70] . For detection of the active forms of Ras, Rac1 or Cdc42 cells were lysed in lysis buffer (50 mM Tris–HCl (pH 7.4), 150 mM NaCl, 5 mM MgCl 2 , 1% Nonidet P-40, 0.5% sodium deoxycholate, 0.1% SDS, 1 mM Na 3 VO 4 ). After centrifugation, the resulting supernatants were incubated for 30 min at 4 °C with glutathione S -transferase (GST) fusion proteins containing the Ras-binding domain of c-Raf-1 or the Cdc42/Rac-interactive binding domain of Pak2. The resulting complexes of GTP-bound GTPases and GST fusion proteins were precipitated with the use of glutathione-Sepharose beads (GE Healthcare), washed twice with lysis buffer and eluted. Alternatively, for detection of active RhoA, cells were lysed in a solution containing 50 mM Tris–HCl (pH 7.4), 150 mM NaCl, 30 mM MgCl 2 , 0.1% Triton X-100, 10% glycerol, 1 mM dithiothreitol, 1 mM phenylmethylsulfonyl fluoride, aprotinin (1 μg ml −1 ), leupeptin (1 μg ml −1 ) and a GST fusion protein containing the RBD of rhotekin. The lysates were clarified by centrifugation, and the complex of GTP-bound RhoA and GST-rhotekin (RBD) was precipitated from the resulting supernatants, washed and eluted. Activated GTPases were then detected by immunoblot analysis with antibodies specific for each protein. Full scans of all immunoblots are supplied in Supplementary Fig. S15 . Fluorescence microscopy Cells were imaged with an Olympus IX-71 microscope equipped with BioPoint MAC5000 excitation and emission filter wheels (Ludl Electronic Products, Hawthorne, NY) and a MicroMAX 512BFT cooled charge-coupled device camera (Princeton Instruments, Trenton, NJ). The following filters were used in this study: XF1071 and XF3075 (Omega Optical, Brattleboro, VT) for CFP; BP470-490 and BP510-550 (Olympus) for GFP and AlexaFluor488; XF1068 and XF3079 (Omega Optical) for yellow fluorescent protein; BP520-550 and BA580IF (Olympus) for ExRed, AlexaFluor546 and AlexaFluor594; and XF1071 and XF3079 for FRET. An XF2034 dichroic mirror (Omega) was used throughout experiments. Cells were illuminated with a 75-W-xenon lamp through a 6% neutral density (ND) filter. Exposure times for 2 × 2 binning were 0.5 s and 30 ms for fluorescence images and differential interference contrast images, respectively. MetaMorph software (Universal Imaging, West Chester, PA) was used for control of the charge-coupled device camera and filter wheels, as well as for analysis of cell-imaging data. FRET imaging and data analysis were performed essentially as described previously [12] , [26] , [32] , [33] . In brief, cells were transfected with vectors for biosensors for 24 h, deprived of serum for 4 h and placed in a chamber on a microscope in which the temperature was maintained at 37 °C. A differential interference contrast image as well as CFP and FRET fluorescence images were recorded every 30 s. After 10–15 min, the cells were infected with PR8. In some experiments, cells were exposed to inhibitors for 30 min before infection. FRET efficiency was calculated as a quotient of background-subtracted FRET and CFP images and was presented in an intensity-modified display mode with MetaMorph software. In the intensity-modified display mode shown here, eight colours from red to blue are used to represent the emission ratio, with the intensity of each colour indicating the mean intensity of FRET and CFP as indicated. Immunofluorescence For immunofluorescence staining, cells were fixed with 3% paraformaldehyde for 15 min at room temperature, permeabilized with 0.1% Triton X-100 in PBS for 4 min at room temperature and then incubated with 1% bovine serum albumin to block nonspecific binding of antibodies. The cells were further incubated with primary antibodies (NP, 1:1,000 dilution; c-Myc, 1:1,000 dilution) overnight at 4 °C, after which immune complexes were detected by incubation for 1 h at room temperature in the dark with AlexaFluor488-, AlexaFluor594- or AlexaFluor647-conjugated secondary antibodies (1:250 dilution). For visualization of actin stress fibres, cells were fixed, permeabilized and then incubated with AlxaFluor594-conjugated phalloidin (1:50 dilution; Invitrogen) for 30 min at 37 °C in the dark. Images were acquired with an FV-10i confocal microscope (Olympus, Tokyo, Japan) or an epifluorescence microscope. Virus internalization and infection assays Cells expressing GFP-Rab7 as a marker of late endosomes or GFP-CLCa as a marker of clathrin-coated vesicles were serum starved in phenol red-free DMEM/F12 for 4 h and incubated with PR8 at an MOI of 10 (prepared by dilution of virus stock in conditioned medium) for 1 h (Rab7) or 30 min (CLCa) at 37 °C. In some experiments, inhibitors were added to culture media before the infection. After fixation, the internalized virus particles were visualized by immunostaining with antibodies to NP. Confocal sections (with a z step of 0.2 μm) were acquired from the bottom to the top of the cells and, after background subtraction, all sections were projected on one image plane to visualize all virus particles simultaneously. Vesicles positive for NP or either Rab7 or CLCa were extracted with the use of the ‘granularity’ module of MetaMorph software, and the co-localization of NP with either Rab7 or CLCa was quantified with the ‘measure co-localization’ function. Of note, during our experimental period, NP co-localization with Rab7 was indicative of viruses that were internalized into cells and reached late endosomes, whereas NP-positive and Rab7-negative granules represent the other fractions of particles, including those localizing in early endosome and those adsorbing on the plasma membrane (but not being internalized). Therefore, a decrease in NP co-localization with Rab7 (and a concomitant increase in NP signal without the co-localization) can be observed when virus internalization is inhibited or delayed. Evaluation of virus internalization by immunoblotting was performed as reported previously [25] . In brief, cells were washed with PBS and incubated with the virus at the indicated MOI diluted in PBS at 4 °C for 60 min. The inoculum was aspirated and cells were washed with PBS (4 °C) three times. Cells were lysed in lysis buffer at indicated time points after a temperature shift to 37 °C and subjected to immunoblotting using anti-M1 and anti-NP antibodies. For analysis of virus infection, serum-starved cells treated with inhibitors or left untreated were infected with PR8 at an MOI of 1 for 4 h at 37 °C, after which replicated virus particles in the nucleus were visualized by immunostaining with antibodies to NP; the fluorescence intensity of NP in the nucleus was measured. Assessment of endocytosis For detection of clathrin-independent and -dependent endocytosis, cells plated on collagen-coated glass-bottom dishes (35-mm-diameter; Asahi Techno Glass, Tokyo, Japan) were incubated with AlexaFluor-conjugated dextran (500 μg ml −1 ) and transferrin (500 μg ml −1 ) for 10 min at 37 °C, respectively, followed by extensive washing with PBS (dextran) or by PBS/HCl (pH 3.0, transferrin) to remove the non-internalized substances. Visualized vesicles were extracted with the use of the ‘granularity’ function of MetaMorph software and their fluorescence intensity was quantified. RNA interference siRNAs targeting murine ROCK1 or ROCK2 mRNAs (siROCK1#1: Mm_Rock1_1, siROCK1#2: Mm_Rock1_4, siROCK2#1: Mm_Rock2_2, siROCK2#2: Mm_Rock2_3) were obtained from Qiagen (Valencia, CA) and were introduced into cells by transient transfection with the use of the HiPerFect reagent (Qiagen). AllStars Negative Control siRNA (Qiagen) was used as a control. RNA isolation and quantitative reverse transcriptase–PCR analysis The total RNA was isolated from cells using an RNeasy Mini Kit (Qiagen) according to the manufacturer’s instructions. First-strand cDNA was synthesized from 1.0 μg of total RNA by SuperScript III reverse transcriptase (Invitrogen). Quantitative PCR analysis was performed with the use of a StepOne real-time PCR system (Applied Biosystems, Foster City, CA) and the following primers: ROCK1-F, 5′-GGTATCGTCACAAGTAGCAGCATCA-3′; ROCK1-R, 5′-TAAACCAGGGCATCCAATCCA-3′; ROCK2-F, 5′-TTGCCAACAGTCCCTGGGTAG-3′; ROCK2-R, 5′-CGCCTGGCATGTACTCCATC-3′; GAPDH-F, 5′-AAGGGCTCATGACCACAGTC-3′; and GAPDH-R, 5′-GGATGCAGGGATGATGTTCT-3′. Data were normalized by the corresponding abundance of glyceraldehyde-3-phosphate dehydrogenase (GAPDH) cDNA and then expressed relative to this value for control cells. Statistical analysis For data presented as box-and-whisker plots, the highest and lowest boundaries of the box represent the 25th and 75th percentiles, respectively, and the whiskers above and below the box designate the 5th and 95th percentiles, respectively; the line within the box indicates the median value. Such data were obtained from three independent experiments. Other data are presented as means±s.d. from three independent experiments, each performed in triplicate. Statistical analysis was performed by one-way analysis of variance followed by Student’s t -test. How to cite this article: Fujioka, Y. et al. A Ca 2+ -dependent signalling circuit regulates influenza A virus internalization and infection. Nat. Commun. 4:2763 doi: 10.1038/ncomms3763 (2013).